Bioinspired copper catalyst effective for both reduction and evolution of oxygen In many green electrochemical energy devices, the conversion between oxygen and water suffers from high potential loss due to the difficulty in decreasing activation energy. Overcoming this issue requires full understanding of global reactions and development of strategies in efficient catalyst design. Here we report an active copper nanocomposite, inspired by natural coordination environments of catalytic sites in an enzyme, which catalyzes oxygen reduction/evolution at potentials closely approaching standard potential. Such performances are related to the imperfect coordination configuration of the copper(II) active site whose electron density is tuned by neighbouring copper(0) and nitrogen ligands incorporated in graphene. The electron transfer number of oxygen reduction is estimated by monitoring the redox of hydrogen peroxide, which is determined by the overpotential and electrolyte pH. An in situ fluorescence spectroelectrochemistry reveals that hydroxyl radical is the common intermediate for the electrochemical conversion between oxygen and water. In the discharging process of green electrochemical devices like fuel cells or metal-air batteries, the output energy capacity is mainly determined by the cathodic oxygen reduction reaction (ORR). Great kinetic loss stemming from this sluggish reaction constitutes the main voltage drop as compared with the ones from the anode process, mass transport and ohmic resistance [1] . In principle, ideal catalysts for ORR should have the capability to efficiently break the O=O double bond (enthalpy change of 498 kJ mol −1 ; ref. 2 ). Platinum (Pt) based materials could meet this requirement. However, they are too scarce to realize widespread use, which thus results in another challenging issue that the consumption of Pt is required to be <0.2 g kW −1 above the cell voltage of 0.65 V (ref. 3 ). Therefore, various alternatives have been proposed, mainly including two categories of doped carbonaceous materials [4] , [5] and late transition metals (that is, Mn, Fe, and Co; refs 6 , 7 , 8 ) in different chemical forms. In reality, fewer materials become available since both the activity and electrolyte corrosion at high potentials have to be considered under the extreme environments of the cathode. Especially, in acidic solutions, most of transition metals and their oxide derivatives are not thermodynamically stable, which is a major obstacle for catalysts developments [9] . The analogous situation also exists in the reverse process of oxygen evolution reaction (OER), which is significant for the applications of battery charging and hydrogen fuel production. This process is thermodynamically not favoured. The OER catalysts should be able to overcome both the activation energy barrier ( E a ) and the standard free energy change (Δ G 0 =1.23 eV). The catalytic activity in heterogeneous process is mainly governed by the adsorption enthalpy ( H ads ) of the substrate on catalysts as understood from the volcano plots [10] . The champion activity requires H ads to be controlled in a specific range, since higher H ads will block the followed elemental steps by forming stable intermediates; while lower H ads cannot effectively activate the substrate, which makes the adsorption as the rate limiting step. For transition metals, their H ads values essentially rely on the energetic states of d -electrons, as many works suggested that the catalytic activity varied with the electron energies tuned by the foreign orbitals with alloying [11] , [12] , coordination [13] , [14] and oxidation [15] . According to the crystal field approach, d -orbitals in such processes are rearranged into t 2g - and e g -orbitals. The e g -electrons are more energetic to be paired. The quantitative conclusion proposed by Gasteriger and co-workers [16] , [17] well reflects this fact, which shows that e g -electrons≈1 is optimal for catalysis by studying a series of intrinsic perovskite materials. On the other side, the Faradaic processes involving O 2 usually proceed with multi elemental steps as generally accepted. Previous density functional theory calculation showed that the oxygen containing intermediate (OCI) involved in ORR affected the global catalytic process [18] . Using a simplified dissociation/association mechanism, the higher activity of Pt over other metals can be explained since the energetic conditions of OCI on this metal surface are moderate for realizing multistep reactions, meeting the volcano relationship. In reality, the diversity of OCI makes ORR more complicated and the identification of these intermediates within their short lifetimes is a tough challenge using available analysis techniques. Up to now, both the global ORR and OER processes have not been fully understood yet. Despite, the volcano plots establish a brief relationship between activity and metal properties, they are still not powerful enough for guiding catalyst design as the detailed adsorption behaviours of OCI are not clarified. For ORR, the ideal catalysts may be inspired from the biological systems in nature. The typical examples are cytochrome c oxidase and laccase, their active sites contain the similar metal clusters of assembled Cu 2+ complexes [19] , [20] . Previous work showed that laccase in vitro is more desirable as the quasi-champion potential (onset at 1.2 V versus reversible hydrogen electrode (RHE), pH=4) is observed on its modified electrode [21] , suggesting that Cu 2+ ion is supposed to be an ideal catalytic site as long as the energy level of the d -electrons is tuned to a reasonable state. However, directly mimicking the Cu 2+ complexes as in enzyme might not be a reasonable strategy, by which the achieved activity is clearly not as good as the natural state [22] , [23] . Low overpotential and high reaction rate are hard to be simultaneously achieved [22] . The main reasons for this inefficient catalysis can be ascribed to the absence of appropriate mediators for sequential electron transfer by specific amino-acid chains in apo-enzyme components and the steric variation of the coordination structures after the complexes are assembled on the electrode. Thus, developing a proper strategy to utilize the catalytic ability of Cu 2+ ion remains a challenge. In this work, we propose an effective approach to tune the d -electron density of Cu 2+ active site and simultaneously increase electron transfer rate via the synergistic effect of electronic connection between Cu 2+ and N, and between Cu 2+ and metallic Cu (Cu 0 ) in graphene formed by pyrolysis. Impressive ORR performance on the resultant catalyst is achieved in acidic and alkaline media. Especially, in the latter case, superior activity than commercial Pt/C catalyst is observed with an onset potential of 0.978 V versus RHE. Interestingly, the resultant catalyst also shows the excellent activity towards OER with the onset potential closely approaching the standard potential. The catalytic process has been probed by using electrochemical methods and in situ fluorescence spectroelectrochemistry, and the results imply the importance of overcoming the same energy barrier for HO · generation during ORR and OER. Structural analysis The catalysts were prepared from the pyrolysis of the mixture of graphene oxide (GO) and Cu 2+ -1,10-phenathroline (Cu(phen) 2 ) at different temperature, and labelled as CPG- t ( t denotes the pyrolysis temperature). After pyrolysis, GO as the support of the catalytic sites is converted into graphene, which greatly increases the conductivity of the resultant materials. The typical morphology of CPG-900 was characterized by transmission electron microscopy (TEM, Fig. 1a ). It can be identified that both the basal plains and edges of graphene are coated with heavier nanoparticles as revealed by the darker and discrete regions. The energy dispersive X-ray spectroscopy of the imaged region shows the presence of Cu and N elements ( Supplementary Fig. 1 ). The high resolution TEM image identifies the lattice spacing in one of the nanoparticles as ~0.202 nm ( Fig. 1b ). The fringes revealed by the X-ray diffraction (XRD) pattern are assigned to the Cu (111) crystal face of 2 θ =43.3°. Combining with the coexisted diffractions at 50.5° and 74°, the existence of Cu 0 is confirmed in CPG-900 (ref. 24 ), which infers that the Cu 2+ ions can be reduced via the dehydrogenation of 1,10-phenanthroline ( Fig. 1c ). The composition of CPG-900 was further determined by X-ray photoelectron spectroscopy (XPS), where the total atomic percentage of Cu is measured to be ~3.6% ( Supplementary Fig. 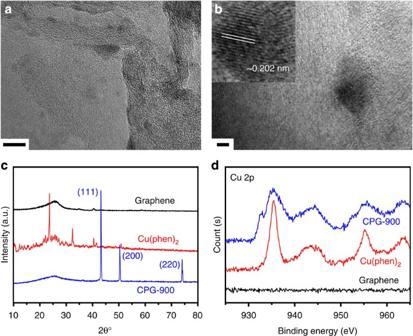Figure 1: Characterizations of CPG-900. Low (a) and high (b) resolution TEM images of CPG-900. The XRD patterns (c) and Cu 2p XPS survey (d) of pristine graphene, Cu(phen)2and CPG-900. Scale bars, 10 nm (a) and 2 nm (b). 2 and Supplementary Table 1, that is, mass percentage of Cu approaching 15%). In the Cu 2p survey, both the 2p 3/2 and 2p 1/2 bands are broadened compared with that of the Cu(phen) 2 precursor, indicating continuum of states for Cu species in CPG-900 ( Fig. 1d ). According to the results from the XRD patterns, the shoulder signals at binding energies of 932.7 and 952.5 eV are attributed to Cu 0 . The main signals at higher binding energies of 935.4 and 955.2 eV are originated from the desired Cu 2+ ions in Cu 2+ –N bond because, (i) the presence of Cu 2p satellites (944.3 and 963.4 eV) demonstrates the unfilled electron state of Cu 3d 9 orbitals [25] ; (ii) the possible composition of copper oxide is excluded from the TEM and XRD results. The result of the broadening characters of Cu 2p are speculated as the coexistence of Cu 0 species and Cu 2+ ions connected to the N atoms with different configurations in graphene. The deoxygenation process of GO allows N doping by replacing some active oxygen atoms. In the N 1 s spectra, the signal band for Cu(phen) 2 precursor split into three after pyrolysis, reflecting the different N configurations (for example, pyridine- and pyrrole-like species). Meanwhile, the Cu 2+ –N–C connection is partially preserved during the N doping process as the binding energies of N 1s at 398.6 and 400.9 eV are coincident with the values reported previously [26] . ( Supplementary Fig. 3 ) The Raman scattering spectra of CPG-900 show several bands as in the case of Cu(phen) 2 precursor at low wavenumbers. The Cu 2+ -N vibration shifts to lower wavenumber of 277 cm −1 for CPG-900 as compared with the one (299 cm −1 ) for Cu(phen) 2 , demonstrating the change of the ligand’s environment ( Supplementary Fig. 4 ) [27] . Figure 1: Characterizations of CPG-900. Low ( a ) and high ( b ) resolution TEM images of CPG-900. The XRD patterns ( c ) and Cu 2p XPS survey ( d ) of pristine graphene, Cu(phen) 2 and CPG-900. Scale bars, 10 nm ( a ) and 2 nm ( b ). Full size image ORR activity and catalytic processes By rotating ring-disk electrode (RRDE) measurements, the current densities of ORR and apparent electron transfer number ( n ) are summarized in Fig. 2a–d . It is found that the pyrolysis temperature plays an important role in determining ORR activity. Among the CPG- t catalysts prepared at pyrolysis temperature ranging from 600–950 °C, the CPG-900 sample shows the optimum result. The Raman scattering spectra show that the intensity ratio of D-band to G-band increases with the pyrolysis temperature, possibly suggesting the gradual incorporation of Cu 2+ -N structure into the graphene forming active sites ( Supplementary Fig. 5 ). In 0.5 M H 2 SO 4 solution saturated with oxygen, the onset potential of ORR appears at 0.855 V versus RHE on CPG-900 and the Tafel slope at low overpotentials is fitted as 71 mV per decade, closely approaching the commercial Pt/C catalyst (66 mV per decade, Fig. 2e ). The current density is, however, not high under the present conditions. This could indicate that the Cu(phen) 2 precursor changes the thermal expansion processes of GO during pyrolysis (that is, generating CO or CO 2 ) [28] , resulting in the low specific surface area of the resultant CPG-900. Nevertheless, the CPG-900 in 0.1 M KOH exhibits the superior activity towards ORR over the commercial Pt/C catalyst as evidenced by both the higher current density and onset potential (0.978 V versus RHE). The Tafel plots show the smaller slope of 49 mV per decade ( Fig. 2f ). Combining with the higher reduction potential, the larger exchange current density on CPG-900 can thus be estimated in the early stage of ORR (ref. 29 ). As expected, the CPG-900 shows little cross effect from methanol oxidation and good CO tolerance as compared with the Pt/C catalyst ( Supplementary Fig. 6 ). In addition, the long-term performance test reveals that the CPG-900 exhibits much better stability than the Pt/C catalyst ( Supplementary Fig. 7 ). The N 2 adsorption/desorption isotherms demonstrate the slight variation of BET surface area (from 79.6–76.2 m 2 g −1 ) and inner pore distribution of the CPG-900 after the stability test and the XPS characterizations confirm the remaining Cu 2+ and Cu 0 components in the catalyst except a minor shift in the binding energy for Cu 2p (that is, 0.3 eV for Cu 2p 3/2 , Supplementary Fig. 8 ). 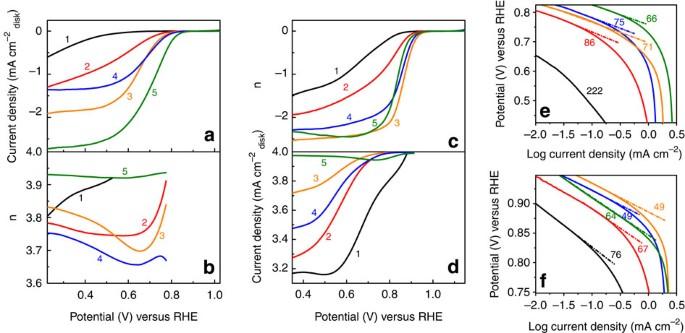Figure 2: ORR catalysis on CPG-900. ORR polarizations (a,c) and correspondingn(b,d) of the CPG-tcatalysts prepared with the pyrolysis temperature of 600 °C (1), 800 °C (2), 900 °C (3) and 950 °C (4) and the corresponding results for the 20% Pt/C catalyst (5) are displayed for comparison. The electrolytes were O2saturated 0.5 M H2SO4(a,b) and 0.1 M KOH (c,d). Rotating speed: 1,000 r.p.m., scan rate: 10 mV s−1. (e,f) The Tafel plots are derived respectively from the data inFig. 1a,c. Figure 2: ORR catalysis on CPG-900. ORR polarizations ( a , c ) and corresponding n ( b , d ) of the CPG- t catalysts prepared with the pyrolysis temperature of 600 °C (1), 800 °C (2), 900 °C (3) and 950 °C (4) and the corresponding results for the 20% Pt/C catalyst (5) are displayed for comparison. The electrolytes were O 2 saturated 0.5 M H 2 SO 4 ( a , b ) and 0.1 M KOH ( c , d ). Rotating speed: 1,000 r.p.m., scan rate: 10 mV s −1 . ( e , f ) The Tafel plots are derived respectively from the data in Fig. 1a,c . Full size image A recent report [30] suggested that ORR could be mediated by the redox of metal active sites existing in the catalysts. This mechanism is not operative in the present study since there is no direct correlation between the redox potential of Cu 2+ ions and ORR potential as indicated by the cyclic voltammogram ( Supplementary Fig. 9 ) and differential pulse voltammogram ( Supplementary Fig. 10 ). To explore the catalytic mechanism of CPG-900, Cu species was leached by HNO 3 treatment. This process increases the BET surface area (from 79.6–128.1 m 2 g −1 , Supplementary Fig. 11 ) and produces more inner micropores, accompanied with the disappearance of Cu signals in TEM images, XRD patterns and Raman scattering spectra ( Supplementary Fig. 12 ). The leached Cu accounts for ~13.3% (mass ratio) of CPG-900 sample as measured by atomic absorption spectroscopy, which is in agreement with the XPS result. The N atomic content of HNO 3 -treated CPG-900 slightly increases due to the physically attached HNO 3 on graphene ( Supplementary Table 2 ). However, the binding energies of these N species shift to lower values, indicating the positively charged Cu 2+ ions detached from the N ligand ( Supplementary Fig. 13d ). As expected, HNO 3 treatment brings significant degradation in the catalytic activity of GPG-900 towards ORR. As shown in Fig. 3a–d , the half-wave potential ( E 1/2 ), reduction current and n greatly decrease in both 0.5 M H 2 SO 4 and 0.1 M KOH. Thus, it can be reasonably inferred that, (i) the Cu 2+ ions in CPG-900 act as the catalytic sites since HNO 3 -treated CPG-900 sample becomes less active for ORR and Cu 0 is known to be inert towards ORR. The observed catalysis of HNO 3 -treated CPG-900 is from the remaining Cu 2+ ions ( Supplementary Fig. 13 ), and the catalytic current can be enhanced by re-coordinating more Cu 2+ ions into the residual N ligands doped in graphene ( Supplementary Fig. 14 ); (ii) Cu 2+ ions are both connected with the N ligand and surface Cu 0 of Cu nanoparticles ( Fig. 3e ). The coordination of N to Cu 2+ ions should not be as perfect as that in the case of the Cu(phen) 2 precursor due to the steric rigidity of graphene structure and nanoparticle. Such imperfect coordination environments undoubtedly changes the spatial position of O 2 adsorption on Cu 2+ ions, which might be more close to mimic the ones of the Cu 2+ centre in laccase; (iii) after pyrolysis, the electron donating ability of N ligand becomes weaker as the electron pairs are conjugated by the π -electrons of graphene [30] as well as the imperfect coordination configurations. In addition, the Cu 0 can donate electrons to the connected Cu 2+ ions as indicated by the slight shift of the binding energy of Cu 2p ( Fig. 1d ). X-ray absorption spectroscopy ( Fig. 3f ) measurements show a sharp band of the 2p 3/2 to 3d transition of Cu 2+ ions in CPG-900 at 930.1 eV, which is lower than Cu(phen) 2 , but higher than Cu(Ac) 2 . This result indicates that the electron donating ability of Cu 0 seems to be relatively moderate, but is still stronger than the 1,10-phenanthroline ligand. (iv) The extended X-ray absorption fine structure measurements of the Cu K -edge in CPG-900 exhibit the typical Cu nanocrystalline features. In the derived oscillation spectra, the amplitude of CPG-900 is whereas smaller than that of Cu foil, indicating the structural defects in Cu nanoparticle due to the size effect ( Supplementary Fig. 15 ). The surface Cu 0 atoms should provide the free electrons to fill the d -orbitals of Cu 2+ ions via dangling bonds. A similar phenomenon has been reported that the Au 1+/3+ ions, which are stable on the Au 0 /CeO 2 nanoparticle system, function as the active sites for catalysis [31] . Thereby, the synergistic electronic effect from Cu 0 and N ligands should make a preferable bonding between O 2 and Cu 2+ ions. This configuration is distinctly different from the cases for the neighbouring transition metals (that is, Fe/Co 2+ coordination structure) [8] , [30] , [32] . The present results reflect that the catalytic activity of transition metals is governed by both the electron arrangement of metal centres and its coordination surroundings. 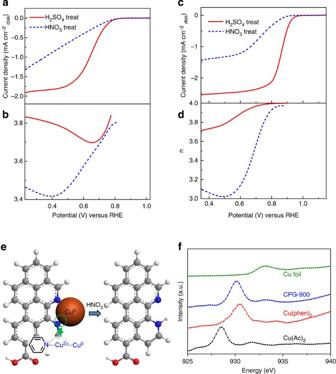Figure 3: Active sites in CPG-900. ORR polarizations (a,c) and correspondingn(b,d) obtained on CPG-900 before and after treated with HNO3in O2saturated 0.5 M H2SO4(a,b) and 0.1 M KOH (c,d). Rotating speed: 1,000 r.p.m., scan rate: 10 mV s−1. (e) Schematic illustration shows the proposed active sites in CPG-900. (f) XAS characterizations of the CuL3-edge in Cu(Ac)2, Cu(phen)2, CPG-900 and Cu foil. Figure 3: Active sites in CPG-900. ORR polarizations ( a , c ) and corresponding n ( b , d ) obtained on CPG-900 before and after treated with HNO 3 in O 2 saturated 0.5 M H 2 SO 4 ( a , b ) and 0.1 M KOH ( c , d ). Rotating speed: 1,000 r.p.m., scan rate: 10 mV s −1 . ( e ) Schematic illustration shows the proposed active sites in CPG-900. ( f ) XAS characterizations of the Cu L 3 -edge in Cu(Ac) 2 , Cu(phen) 2 , CPG-900 and Cu foil. Full size image It is clear that the n of ORR strongly depends on the overpotential and electrolyte pH. In the RRDE experiments, the n is governed by the ratio of the H 2 O 2 oxidation reaction current on ring to that of ORR current on disk. Although the reactions of H 2 O 2 on the disk electrode are usually neglected, they surely affect both the ring and disk currents ( Fig. 4a ). As generally accepted, the reaction rates of H 2 O 2 are determined by its adsorption/desorption processes [33] , [34] . At open circuit potential, the influence of H 2 O 2 decomposition on the RRDE results is estimated to be rather limited ( Supplementary Fig. 16 ). While within the potentials for ORR, the redox behaviours of H 2 O 2 are involved on CPG-900, which closely correlate to the n of ORR. As shown in Fig. 4b , in the early stage of ORR (0.5 M H 2 SO 4 , A zone), H 2 O 2 is reoxidized to O 2 on the disk electrode, which reflects moderate adsorption energy of H 2 O 2 on CPG-900. Thus, a more favoured H 2 O 2 decomposition is also expected on CPG-900 comparing to that at open circuit potential. These processes result in much less H 2 O 2 detected on the ring electrode and higher n (4-3.8). In the following stage (B zone), the redox of H 2 O 2 appears to be relatively slow, showing that the desorption of H 2 O 2 from CPG-900 becomes dominant, thus, more H 2 O 2 is detected on the ring electrode and the n gradually reaches the minimum of 3.7. At more negative potentials (C zone), the n arises due to the contribution from the H 2 O 2 reduction reaction (HRR). On the other hand, the n of ORR continuously decreases with increasing the overpotential in 0.1 M KOH ( Fig. 4c ). In this case, only two zones (A and B) in the relationship between n and overpotential appear due to the absence of fast reduction of H 2 O 2 process. In A zone, H 2 O 2 is not detected at the ring electrode since all the formed H 2 O 2 during ORR is reoxidized to O 2 or/and decomposed, and thus, the n keeps as 4. This result benefits for the terminal fuel cell assembly because the transient state of ORR is used to assess the half-cell voltage, where the catalytic current and overpotential reach balanced [3] . With the increase of overpotential, the n decreases continuously from 4 to 3.7, reflecting that the H 2 O 2 reduction and/or decomposition gradually become trivial comparing to the desorption of H 2 O 2 from CPG-900. 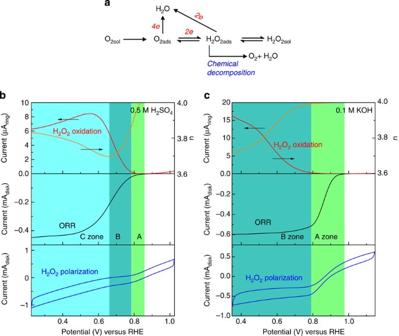Figure 4: Influence of H2O2adsorption/desorption onnof ORR. (a) Schematic illustration of the different reaction pathways of H2O2involved in ORR (the subscripts of ‘sol’ and ‘ads’ stand for the reaction species dissolved in bulk solution and adsorbed on CPG-900, respectively). The polarization curves of 5 mM H2O2on CPG-900 in 0.5 M H2SO4(b) and 0.1 M KOH (c) was characterized using cyclic voltammetry at a rotating rate of 1,000 r.p.m., 10 mV s−1in N2atmosphere. ORR current, H2O2oxidation reaction (HOR) current andnin O2saturated electrolyte are all summarized in the same figure, aiming to explain the relationships ofnversus overpotential. Figure 4: Influence of H 2 O 2 adsorption/desorption on n of ORR. ( a ) Schematic illustration of the different reaction pathways of H 2 O 2 involved in ORR (the subscripts of ‘sol’ and ‘ads’ stand for the reaction species dissolved in bulk solution and adsorbed on CPG-900, respectively). The polarization curves of 5 mM H 2 O 2 on CPG-900 in 0.5 M H 2 SO 4 ( b ) and 0.1 M KOH ( c ) was characterized using cyclic voltammetry at a rotating rate of 1,000 r.p.m., 10 mV s −1 in N 2 atmosphere. ORR current, H 2 O 2 oxidation reaction (HOR) current and n in O 2 saturated electrolyte are all summarized in the same figure, aiming to explain the relationships of n versus overpotential. Full size image Stepwise electron transfer of ORR It is assumed that OCI is involved in the ORR. However, verifying such assumption is rather difficult as the lifetime of OCI is quite short in aqueous media, especially within the interface layer with applied electrical field [35] , [36] . To solve this issue, we applied in situ fluorescent spectroscopy combining with electrochemical techniques to probe the formation of OCI using 2′,7′-dichlorodihydrofluorescein (DCDHF) as an indicator [37] . Upon reacting with the OCI generated in ORR, DCDHF will be converted to fluorescent dichlorofluorescein (DCF, Fig. 5a ). As shown in Fig. 5b , during ORR at 0.848 V versus RHE (the cathodic current is about −20 μA), an emission at 522 nm continuously grows with electrolyzing time in 0.1 M KOH containing 2.5 μM DCDHF. To verify the detected OCI is a transient state rather than a byproduct, ORR on CPG-900 was performed at 0.849 V versus RHE in a solution of 0.01 M KOH in 1:1 (v/v) water/ethanol solvent saturated with air. A distinct decrease in the reduction current occurs upon addition of DCDHF ( Fig. 5c ), demonstrating that the formation of OCI is followed by an electrochemical reaction that it can further receive electron from electrode to accomplish the ORR and a parallel chemical reaction with DCDHF to form fluorescent DCF. The appearance of the fluorescence emission from H 2 O 2 can be ruled out as no significant fluorescence emission is observed when 8 μM H 2 O 2 is solely added into 0.1 M KOH without applying potential ( Supplementary Fig. 17 ). Further experiments identified the observed OCI as HO · radical by using a specific signal molecule, coumarin. As shown in Fig. 5d , the fluorescence emission at 500 nm increases due to the hydroxylation of coumarin seventh position during the ORR. This result agrees with the observation acquired on a Pt electrode [38] . 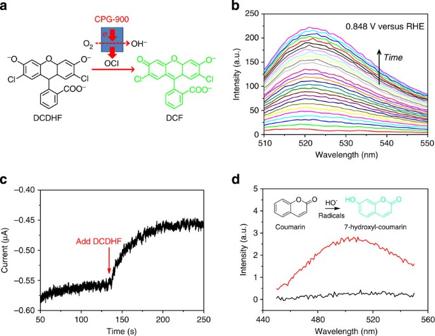Figure 5: Probing the multi elemental steps of ORR. (a) Schematic illustration of the conversion from non-fluorescent DCDHF to fluorescent DCF by the OCI formed in ORR on CPG-900. (b)In situfluorescence spectroelectrochemistry performed at a constant potential in O2saturated 0.1 M KOH containing 2.5 μM DCDHF for 10 min (from bottom to top). (c)I–Tcurve of ORR on CPG-900 at 0.849 V versus RHE. The electrolyte is 0.01 M KOH dissolved in 1:1 (v/v) water/ethanol solution with saturated air. The red arrow denotes the addition of 12.5 μM DCDHF into the electrolyte, showing an abrupt decrease in reduction current due to the competitive chemical reaction of OCI with DCDHF to the electrochemical reaction by receiving electrons from CPG-900. (d)In situfluorescence spectroelectrochemistry performed at 0.799 V versus RHE with 60 μM coumarin to specifically verify the presence of HO·radicals. To avoid the hydrolysis of ester ring in coumarin, the electrolyte was diluted to be 0.01 M KOH saturated with O2(refs39,40). The electrolysis lasted for ~50 min (the black and red lines stand for the initial and final signals, respectively). Figure 5: Probing the multi elemental steps of ORR. ( a ) Schematic illustration of the conversion from non-fluorescent DCDHF to fluorescent DCF by the OCI formed in ORR on CPG-900. ( b ) In situ fluorescence spectroelectrochemistry performed at a constant potential in O 2 saturated 0.1 M KOH containing 2.5 μM DCDHF for 10 min (from bottom to top). ( c ) I – T curve of ORR on CPG-900 at 0.849 V versus RHE. The electrolyte is 0.01 M KOH dissolved in 1:1 (v/v) water/ethanol solution with saturated air. The red arrow denotes the addition of 12.5 μM DCDHF into the electrolyte, showing an abrupt decrease in reduction current due to the competitive chemical reaction of OCI with DCDHF to the electrochemical reaction by receiving electrons from CPG-900. ( d ) In situ fluorescence spectroelectrochemistry performed at 0.799 V versus RHE with 60 μM coumarin to specifically verify the presence of HO · radicals. To avoid the hydrolysis of ester ring in coumarin, the electrolyte was diluted to be 0.01 M KOH saturated with O 2 (refs 39 , 40 ). The electrolysis lasted for ~50 min (the black and red lines stand for the initial and final signals, respectively). Full size image Extended application for OER The catalytic process of OER on CPG-900 is also analyzed by RRDE method to avoid the influence from produced bubbles ( Fig. 6a ). The obtained onset potential closely approaches the standard potential, as low as 1.34 V (in 0.1 M KOH) and 1.23 V (in 0.5 M H 2 SO 4 ) versus RHE, which are superior to many OER catalysts reported recently ( Supplementary Table 3 ). Being analogous to ORR, the selectivity of OER is studied by recording the ring current at a potential with respect to the H 2 O 2 oxidation. In 0.5 M H 2 SO 4 , a much smaller anodic current at the ring electrode (1/5,000~1/2,500 of the disk current) occurs, suggesting that the global OER is almost a 4e -transfer but is still involved with trace amount of the H 2 O 2 byproduct. Interestingly, in 0.1 M KOH, a relatively small and cathodic ring current is observed although the ring electrode potential is kept more positive for H 2 O 2 oxidation ( Fig. 6b ). At 1.348 V versus RHE, the reduction behaviours of O 2 , H 2 O 2 or H 2 O on the Pt ring electrode are rather impossible. The observed cathodic ring current is more likely originated from the reduction of OCI. Thereby, the OER is probed by the in situ fluorescence spectroelectrochemistry. Using DCDHF indicator, the fluorescence emission at 522 nm keeps increasing at an anodic current of 3–4 μA, demonstrating that the OCI is exactly involved in OER ( Fig. 6c and Supplementary Fig. 18 ). 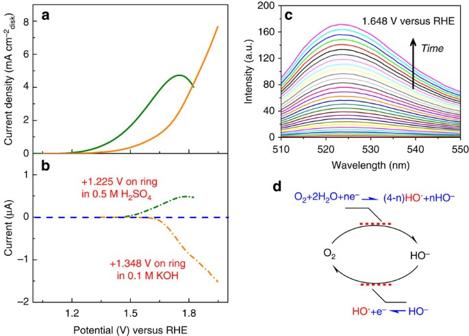Figure 6: A brief correlation between ORR and OER. OER polarizations (a) and corresponding ring currents (b) obtained on CPG-900 in 0.5 M H2SO4(olive line) and 0.1 M KOH (orange line). Rotating speed: 1,000 r.p.m., scan rate: 10 mV s−1. (c)In situfluorescence spectroelectrochemistry performed at constant potential in 0.1 M KOH containing 2.5 μM DCDHF. (d) Schematic illustration of the electrochemical conversion between O2and HO−, which experiences a common transient state of HO·radical. Figure 6: A brief correlation between ORR and OER. OER polarizations ( a ) and corresponding ring currents ( b ) obtained on CPG-900 in 0.5 M H 2 SO 4 (olive line) and 0.1 M KOH (orange line). Rotating speed: 1,000 r.p.m., scan rate: 10 mV s −1 . ( c ) In situ fluorescence spectroelectrochemistry performed at constant potential in 0.1 M KOH containing 2.5 μM DCDHF. ( d ) Schematic illustration of the electrochemical conversion between O 2 and HO − , which experiences a common transient state of HO · radical. Full size image According to the above results, the most possible OCI in OER could be O 2 − and HO · radicals. But injecting electrons to O 2 − consumes too much energy. In contrast, the elemental reaction (HO · to HO − , E 0 =1.9 V versus standard hydrogen electrode [38] ) is more energetically favourable, which can reasonably explain the origin of the reduction event on the Pt ring in 0.1 M KOH. Using coumarin indicator, the presence of HO · radicals is confirmed by the increased fluorescence emission at 500 nm ( Supplementary Fig. 19 ). Accordingly, we establish a brief relationship between ORR and OER. With respect to the standard potential of HO · radical, the overpotential for both ORR and OER should be at least 1.25 V (O 2 +2H 2 O+ne − →(4−n)HO · +nHO − E 0 =−0.024 V versus standard hydrogen electrode [38] ). The actual energetic state of this specie on the CPG-900 surface is altered, which would be a major reason to decrease the overpotentials of OER and ORR in alkaline solutions ( Fig. 6d ). In addition, OER is normally not thermodynamically favoured. But in the present study, the observed overpotential of OER is lower than ORR, suggesting that the initial adsorption of HO − and O 2 on CPG-900 is different. The more favourable bonding configuration might be the adsorption of polarized HO − on Cu 2+ ions. In summary, a high performance Cu nanocomposite (CPG-900) is synthesized by the pyrolysis of the mixture of GO and Cu(phen) 2 as inspired by the catalytic sites in natural enzyme. The electron density of Cu 2+ active sites in CPG-900 is tuned by the electron donation effect from both the neighbouring Cu 0 of Cu nanoparticle and the N ligand incorporated in the rigid graphene. This imperfect coordination configuration provides an optimal environment for electronic bonding of O 2 to Cu 2+ ions. The ORR occurs on the CPG-900 with overpotential of only ~0.25 V in 0.1 M KOH, referencing to the standard potential. Since the reactions of H 2 O 2 involve in the ORR process, the n of ORR varies with the overpotential and electrolyte pH. In addition, the CPG-900 shows excellent catalytic activity towards OER with the onset potential approaching the standard potential. Results from the in situ fluorescence spectroelectrochemistry measurements establish a brief correlation between ORR and OER in alkaline solutions, showing that both the processes are intermediated by the HO · radical. This work offers a new insight into the OER/ORR mechanism and possible strategies to design high performance catalysts. Reagents Graphite powder (99.9995%, 100 mesh) was purchased from Alfa Aesar Company (UK). Both Cu(Ac) 2 and 1,10-phenathtoline (phen) were purchased from Nanjing Chemical Reagent Co. Ltd (China). Other reagents were of analytical-reagent grade. All aqueous solutions were prepared with Millipore water (resistivity of 18.2 MΩ cm). Synthesis of Cu(phen) 2 -graphene nanocomposite The Cu 2+ -1,10-phenanthroline (Cu(phen) 2 , Supplementary Fig. 20 ) precursor was synthesized by heating the mixed solution of Cu(Ac) 2 (0.5 mmol dissolved in 30 ml dimethyl formamide) and 1,10-phenanthroline (1 mmol dissolved in 70 ml CH 2 Cl 2 ) at 35 °C for 8 h. The solvents of the solution were then removed by rotary evaporation. The remaining solid was successively washed by acetone and CH 2 Cl 2 until turning into emerald. The GO precursor was synthesized via chemical exfoliation of graphite. Briefly, the mixture of graphite (6 g), K 2 S 2 O 8 (3 g) and P 2 O 5 (3 g) were heated at 80 °C for 8 h in concentrated H 2 SO 4 . The as-obtained graphite (2 g) was oxidized by KMnO 4 (6 g) in concentrated H 2 SO 4 at 35 °C for 2 h. The mixture of Cu(phen) 2 and GO was pyrolyzed with a mass ratio of 2:1 in Ar atmosphere, resulting in Cu(phen) 2 -graphene nanocomposites (CPG- t , t denotes the pyrolysis temperature ranging from 600–950 °C). To exclude any unstable phases in acidic media, the pyrolyzed product was treated in H 2 SO 4 (0.5 M) at 80 °C for 2 h before each characterization. In a controlled experiment, the CPG-900 was further treated with HNO 3 (1.3 M) for the leaching of Cu. This process was performed at 80 °C for 2 h in air atmosphere. Afterwards, the HNO 3 solution was removed by centrifugation and the resultant solid product was washed with ethanol several times and finally dried under pressure at room temperature. Apparatus The ultraviolet–visible spectra were obtained on a Nanodrop-2000C spectrophotometer (Thermo Fisher Scientific Company, USA). The electron paramagnetic resonance characterizations were performed on an EMX-10/12 spectrometer (Bruker Company, Germany). The morphologies of each sample were characterized by TEM (JEM-2100, JEOL Company, Japan). The TEM samples were prepared by drying a droplet of sample suspension on Ni-grids with carbon film. The XRD and Raman spectra were carried out on a X'TRA (ARL Company, Switzerland) and a FT-Raman spectrometer (Bruker company), respectively. The XPS were obtained on a PHI 5000 VersaProbe spectrometer (UlVAC-PHI Company, Japan). The curve fitting of elemental fine spectra was performed using 20% Gaussian–Lorentzian peak shape. The atomic absorption spectroscopy was performed for measuring the leached Cu (180-80 type, Hitachi Company, Japan). The hard X-ray absorption experiments at Cu K -edge were performed at room temperature in the transmission mode using a ion chamber detector at beam line BL14W1 of the Shanghai Synchrotron Radiation Facility (SSRF), China. The photon energy was calibrated with the first inflection point of Cu K -edge in Cu foil. The soft X-ray absorption experiments at Cu L -edge were performed at beam line BL08U. During the measurements, the synchrotron was operated at an energy level of 3.5 GeV and a current between 150–210 mA. Electrochemical measurements A glassy carbon (GC, 5.61 mm in diameter) disk and a Pt (0.84 mm in width) ring were applied as the working electrodes fixed on the rotating apparatus (PINE Company, USA). Prior to electrochemical measurements, the GC disk and Pt ring electrodes were polished with 0.05 μm alumina slurries. Then, the electrodes were successively sonicated in ethanol and deionized water. The Pt ring electrode was further electrochemically polished in 0.5 M H 2 SO 4 . A 6 μl suspension (10 mg ml −l CPG- t sample dispersed in ethanol) was casted on the GC disk and was later covered with a layer of Nafion film while without contacting the Pt ring electrode. The ORR and OER electrochemical measurements were performed on a CHI 900D potentiostat (CH Instrument Company, USA) with Ag/AgCl electrode and Pt wire as reference and counter electrodes, respectively. The onset potential is determined by the value where current starts to show above (OER)/ below (ORR) zero. The collection efficiency ( N ) of the working electrodes modified with catalysts was measured by using 5 mM [Ru(NH 3 ) 6 ] 3+ /0.1 M KCl solution in N 2 atmosphere. The apparent electron transfer number ( n ) of ORR was calculated by the following equation: where, i d stands for the current of ORR on GC disk electrode and i r stands for the current of H 2 O 2 oxidation reaction on Pt ring electrode. The potentials of ORR and OER were converted to the values referring to the RHE. In 0.5 M H 2 SO 4 , the open circuit potential remains at 0.2249 V ( E (RHE)= E (Ag/AgCl)+0.2249 V), rarely showing fluctuation; in 0.1 M KOH, the open circuit potential remains at 0.9482 V ( E (RHE)= E (Ag/AgCl)+0.9482 V), showing slight variation of 0.0001 V ( Supplementary Fig. 21 ). In situ fluorescence spectroelectrochemistry The experiment was designed by combining an electrolysis unit (CHI 660D, CH Instrument Company) with fluorescence spectrophotometer (RF-5301PC, Shimadzu, Japan). Typically, CPG-900 suspension (1 μl) was dropped on GC electrode (3 mm in diameter) in a three-electrode system. The DCDHF (2.5 μM) signal probe was added into 0.1 M KOH before ORR/OER. The stock solution of 1.25 mM DCDHF was prepared using 0.01 M KOH in water/ethanol (1:1, v/v) solvent. During electrolyzing, the OCI involved in ORR/OER instantaneously react with DCDHF, generating fluorescent DCF. Verification of the presence of HO · radicals was performed at room temperature (14 °C estimated by an infrared thermometer) using specific coumarin signal probe. To avoid the hydrolysis of contained ester ring, the concentration of KOH electrolyte was diluted to 0.01 M. With the generation of HO · species, the hydroxylation of coumarin will occur at the seventh position, greatly increasing the fluorescent emission upon excitation at 360 nm. How to cite this article : Wang, J. et al. Bioinspired copper catalyst effective for both reduction and evolution of oxygen. Nat. Commun. 5:5285 doi: 10.1038/ncomms6285 (2014).